Interaction between emotional state and learning underlies mood instability Intuitively, good and bad outcomes affect our emotional state, but whether the emotional state feeds back onto the perception of outcomes remains unknown. Here, we use behaviour and functional neuroimaging of human participants to investigate this bidirectional interaction, by comparing the evaluation of slot machines played before and after an emotion-impacting wheel-of-fortune draw. Results indicate that self-reported mood instability is associated with a positive-feedback effect of emotional state on the perception of outcomes. We then use theoretical simulations to demonstrate that such positive feedback would result in mood destabilization. Taken together, our results suggest that the interaction between emotional state and learning may play a significant role in the emergence of mood instability. What makes you happier, finding a stray dime when in a good mood, or in the middle of a bad day? Outcomes may be subjectively perceived as better when one is in a good mood [1] . But unexpected outcomes can also change one’s mood [2] , [3] . This would result in a positive feedback loop, in which improved outcomes improve mood, which then further improves perceived outcomes. Conversely, good outcomes could devalue subsequent outcomes due to diminishing subjective value (think about finding a dime right after winning the lottery). This latter possibility, which is consistent with prospect theory in behavioural economics [4] , [5] , suggests, in contrast, negative feedback dynamics. While negative feedback typically promotes stability, positive feedback constitutes a principal cause of instability throughout the natural world [6] , [7] , [8] , [9] , [10] , [11] . Accordingly, we hypothesized that individuals with a positive feedback relationship between emotional state and outcomes would tend to suffer from instability of mood, whereas negative feedback would be associated with emotionally stability. We thus set forth to test the effect of a large unexpected outcome on emotional state and on the valuation of subsequent outcomes. Fifty-six human participants played a game in which they chose between pairs of slot machines that differed in probability of dispensing small (25 cent) rewards, learning by trial-and-error which machine is more rewarding ( Fig. 1a ). Then, to induce a change in emotional state, we held a wheel of fortune (WoF) draw in which participants either won or lost a relatively large sum ($7) at chance. Following this, participants played two more slot machine games, each with a new set of slot machines. If an unexpected outcome induces an emotional state, which then feeds back positively onto the perception of outcomes, winning the WoF draw should make participants happier, and, in addition, they should value rewards received after the draw more highly than those received before the draw. Critically, for a positive feedback loop to ensue, subjective valuations must increase above and beyond any shift in reference point that may diminish valuations of subsequent rewards [4] . Similarly, participants who lose the draw should become less happy and value subsequent rewards less highly. 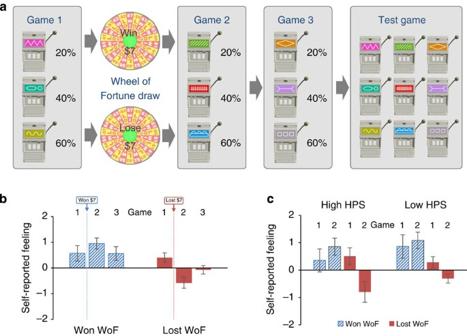Figure 1: Experimental design and emotional response. (a) The experiment included three slot-machine games, a wheel of fortune (WoF) draw, and a test game. Half of the participants won $7 in the WoF draw and half lost $7. In the test phase, participants were asked to choose between slot machines that they had learned about before and after the draw. Reward obtained during the test game was not revealed until the end of the experiment so as to test previously learned valuations of the slot machines. (b) Mean self-reported feeling during the three slot-machine games, on a scale of 5 (completely happy) to −5 (completely unhappy). Winning the WoF draw improved mood, whereas losing the draw had the opposite effect (n=56,t54=4.6,P<10−5,ttest). (c) Mean self-reported feeling during the first and second slot-machine games, as function of HPS score. Participants were divided into equal-sized groups using a median split on HPS score. Participants with higher HPS scores were more strongly affected by the WoF draw (n=56,F1,52=8.5,P=0.005, ANCOVA HPS × WoF interaction). Error bars, s.e.m;n=56 participants, including data from both behavioural and fMRI experiments. Figure 1: Experimental design and emotional response. ( a ) The experiment included three slot-machine games, a wheel of fortune (WoF) draw, and a test game. Half of the participants won $7 in the WoF draw and half lost $7. In the test phase, participants were asked to choose between slot machines that they had learned about before and after the draw. Reward obtained during the test game was not revealed until the end of the experiment so as to test previously learned valuations of the slot machines. ( b ) Mean self-reported feeling during the three slot-machine games, on a scale of 5 (completely happy) to −5 (completely unhappy). Winning the WoF draw improved mood, whereas losing the draw had the opposite effect ( n =56, t 54 =4.6, P <10 −5 , t test). ( c ) Mean self-reported feeling during the first and second slot-machine games, as function of HPS score. Participants were divided into equal-sized groups using a median split on HPS score. Participants with higher HPS scores were more strongly affected by the WoF draw ( n =56, F 1,52 =8.5, P =0.005, ANCOVA HPS × WoF interaction). Error bars, s.e.m; n =56 participants, including data from both behavioural and fMRI experiments. Full size image Our results show that an outcome that affects emotional state also biases the valuation of subsequent outcomes, but only in participants who report a tendency to mood instability. A computational model suggests that such a bidirectional interaction between perceived outcomes and emotional state may, in fact, generate mood instability. The effect of wheel of fortune outcomes on emotional state To evaluate emotional state, at 3 points during each slot-machine game we asked participants to rate how they currently feel. The data indicated that the result of the WoF draw significantly affected participants’ feeling during the subsequent slot-machine game (mean mood change: +0.38±0.24 for participants who won the WoF draw versus −0.97±0.16 for participants who lost the WoF draw, n =56, t 54 =4.6, P <10 −5 , t test), though by game 3 this effect was no longer significant ( n =56, t 54 =1.7, P =0.09, t test, for difference between the third and first games; Fig. 1b ). In addition, the WoF draw resulted in an increase in pupil diameter, indicating increased emotional arousal [12] (mean diameter change across both Win and Lose groups: +4.0%±1.0%, n =45, t 44 =4.1, P <10 −4 , t test; there were no significant differences between the groups or between game 2 and game 3). We therefore focused our subsequent analyses on the first and second game, that is, the games immediately before and immediately after the WoF draw. We next examined whether the degree to which the WoF outcome affected feeling was correlated with susceptibility to mood instability. To this end, participants completed the International Personality Item Pool [13] version of the Hypomanic Personality Scale [14] (HPS)—a self-report measure that has been shown to correlate with frequency of good and bad moods [15] , as well as with risk of developing bipolar disorder [16] . A higher HPS score (indicating less stable mood) was associated with a greater change in feeling following the WoF draw ( Fig. 1c ; n =56, F 1,52 =8.5, P =0.005, ANCOVA HPS × WoF interaction), but accounting for differences in baseline mood level (that is, before the WoF draw) weakened this result to trend level ( n =56, F 1,52 =3.6, P =0.06, ANCOVA HPS × WoF interaction). The effect of the WoF on perception of subsequent outcomes To examine whether the WoF draw affected not only participants’ emotional state, but also their subsequent valuations, in a final test game participants chose between slot machines that had appeared before and after the WoF draw, and had objectively similar reward probabilities ( Fig. 1a ). As predicted, participants with high HPS scores who won the draw favoured slot machines that they had encountered after the draw, whereas participants with high HPS scores who lost the draw favoured slot machines encountered before the draw. In contrast, participants with low HPS scores were not biased by the outcome of the draw. This result was true both for participants who only performed the behavioural experiment ( Fig. 2a ; n =30, F 1,26 =4.1, P =0.05, ANCOVA HPS × WoF interaction), and for a separate group of participants who performed the experiment in a Magnetic Resonance Imaging (MRI) scanner ( Fig. 2b ; n =26, F 1,22 =4.2, P =0.05, ANCOVA HPS × WoF interaction; see Supplementary Fig. 1 for the combined data). Furthermore, this result could not be explained by an effect of the WoF outcome on the balance between exploration and exploitation (see Methods for details). Interestingly, the WoF draw did not bias participants’ explicit valuations of how likely each machine was to yield reward ( n =56, F 1,52 =0.02, P =0.88, ANCOVA HPS × WoF interaction). This is consistent with our hypothesis that the behavioural bias reflected biased perception of the subjective value of reward, not the frequency of reward. 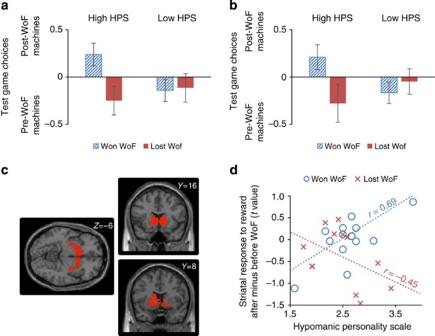Figure 2: Test-game slot-machine choices and striatal response to reward, as a function of HPS score and WoF outcome. (a,b) Difference between percent choices of post-WoF slot machines and pre-WoF slot machines, in the behavioural experiment (a,n=30 participants,F1,26=4.1,P=0.05, ANCOVA HPS × WoF interaction) and in the fMRI experiment (b,n=26,F1,22=4.2,P=0.05, ANCOVA HPS × WoF interaction). (c) A striatal region of interest was defined at the group level as those voxels within the anatomical boundaries of the striatum that responded more to reward than to no-reward outcomes throughout the experiment (P<0.0001 uncorrected, GLM).YandZindicate MNI coordinates. (d) Striatal response to reward in game 2 (which followed the WoF draw) compared with game 1, as a function of HPS (GLM), divided according to the outcome of the WoF draw (totaln=25). HPS scores are on a scale of 1 (least hypomanic) to 5 (most hypomanic). The difference between the Win and Lose groups (F1,21=10.1,P<0.005, ANCOVA HPS × WoF interaction) remained statistically significant when tested using robust regression (t1,21=2.8,P<0.05), indicating that it could not be explained by the effect of outliers. Figure 2: Test-game slot-machine choices and striatal response to reward, as a function of HPS score and WoF outcome. ( a , b ) Difference between percent choices of post-WoF slot machines and pre-WoF slot machines, in the behavioural experiment ( a , n =30 participants, F 1,26 =4.1, P =0.05, ANCOVA HPS × WoF interaction) and in the fMRI experiment ( b , n =26, F 1,22 =4.2, P =0.05, ANCOVA HPS × WoF interaction). ( c ) A striatal region of interest was defined at the group level as those voxels within the anatomical boundaries of the striatum that responded more to reward than to no-reward outcomes throughout the experiment ( P <0.0001 uncorrected, GLM). Y and Z indicate MNI coordinates. ( d ) Striatal response to reward in game 2 (which followed the WoF draw) compared with game 1, as a function of HPS (GLM), divided according to the outcome of the WoF draw (total n =25). HPS scores are on a scale of 1 (least hypomanic) to 5 (most hypomanic). The difference between the Win and Lose groups ( F 1,21 =10.1, P <0.005, ANCOVA HPS × WoF interaction) remained statistically significant when tested using robust regression ( t 1,21 =2.8, P <0.05), indicating that it could not be explained by the effect of outliers. Full size image If biased test-game choices indeed resulted from biased perception of reward, we should expect to see a corresponding bias in neural responses to rewards in the striatum—a brain area where blood-oxygen-level dependent (BOLD) signals have been shown to reflect a reward prediction error signal that drives learning and guides future choices [17] , [18] , [19] , [20] , [21] , [22] , [23] , [24] , [25] ( Fig. 2c ). To test for this, we compared striatal BOLD responses with slot machine rewards before and after the WoF draw. Higher HPS score was associated with stronger BOLD responses to rewards in the second game for participants who won the WoF draw, and weaker responses to rewards for participants who lost the draw ( Fig. 2d ; n =25, F 1,21 =10.1, P <0.005, ANCOVA HPS × WoF interaction). This interaction between HPS score and WoF outcomes was also significant ( n =25, t 1,21 =2.8, P <0.05, robust regression) under a more conservative analysis that accounts for potential outliers [26] , [27] , as well as when controlling for differences in the balance between exploration and exploitation (see methods for details). Moreover, a whole-brain analysis revealed a similar bias in the BOLD response to reward in reward-sensitive areas outside of the striatum, and in particular in the ventromedial prefrontal cortex ( Supplementary Fig. 2 ). However, there was no such bias in the BOLD response to the appearance of task stimuli ( n =25, P >0.05, ANCOVA HPS × WoF interaction; see Methods). Thus, the post-WoF draw bias was not due to a general effect of emotional state on BOLD responses (for example, due to global effects on arousal or attention), but rather was specific to the valuation of reward. In sum, our two experiments showed that in participants whose mood tends to be less stable, a large unexpected outcome affected emotional state, and biased reward perception in the same direction. In contrast, participants with more stable mood showed no such positive feedback interaction between unexpected outcomes (and their associated mood) and valuation of future rewards. A model of the interaction between mood and learning We next formalized the feedback interaction between emotional state and reward perception that was evident in our experiments in a reinforcement-learning model [28] in which positive surprises (prediction errors) improve mood and negative surprises worsen mood (see Methods for model equations). In line with previous work [29] , [30] , ‘mood’ was formalized as a running average of recent outcomes. We note that this implementation allows mood both to change gradually due to the aggregated effect of multiple outcomes as is considered typical for mood, or more rapidly, in response to a single highly significant outcome (as is more characteristic of emotions [31] ). Critically, in our model, the effect of mood on subjective perception of reward was controlled by a parameter f . If f =1 mood does not bias reward perception. With f >1, mood exerts positive feedback. That is, reward is perceived as larger in a good mood and as smaller in a bad mood. Conversely, 0< f <1 corresponds to negative feedback, with reward perceived as smaller in a good mood and as larger in a bad mood. To test the validity of the model, we assessed how well it explained participants’ trial-to-trial choices and self-reported feeling throughout the experiment, as compared with two alternative models: a model in which outcomes do not affect mood (‘no mood’ model) and a model in which outcomes affect mood, but mood does not affect perception of outcomes (‘no mood bias’ model). As shown in Fig. 3a , for participants with high HPS scores, the full model outperformed both the ‘no mood’ model and the ‘no mood bias’ model. This indicates that both the effect of outcomes on mood and the effect of mood on outcomes played a role in determining the behaviour of participants that are susceptible to mood instability. In contrast, in participants with low HPS scores, the modelling results indicated that outcomes affected mood (that is, the mood model outperformed the ‘no mood’ model), but mood not did not significantly affect perception of outcomes (that is, the ‘no mood bias’ model and the full mood model accounted for participants’ behaviour equally well). 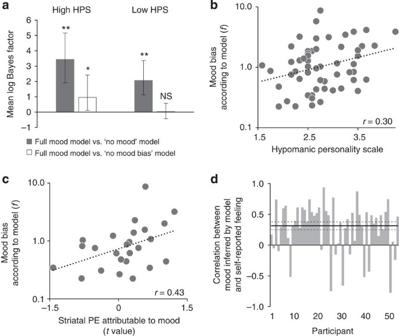Figure 3: Model-based analysis of experimental data using a reinforcement-learning model of mood. (a) Comparison of the mood model to the alternative ‘no mood’ and ‘no mood bias’ models in terms of each model’s ability to explain participants’ behaviour. Positive log Bayes factors favour the full mood model, and negative log Bayes factors favour the alternative model. Participants (n=56) were divided into equal-sized groups using a median split on HPS score. Error bars: bootstrap 95% confidence intervals. **P<10−6, *P<0.05, NS,P>0.5, bootstrap test. (b) Model-estimated mood bias (plotted on a log scale) as compared with HPS score. The more participants were susceptible to mood instability, as measured by the HPS, the more the reward-perception bias inferred by the model tended to the positive (that is, >1;n=56, Pearson’sr=0.3,P<0.05). (c) Participants’ model-estimated mood bias (log scale) was correlated with the degree to which striatal activity followed prediction error signals that are attributable to the effect of mood on perception of reward as compared with standard reinforcement learning prediction errors (n=25, Perason’sr=0.43,P<0.05). Negativet-values reflect anti-correlation between the additional contribution of the positive-feedback model’s mood-induced biases (above and beyond the no-mood model prediction errors) and striatal activations, as would be expected for participants with a negative feedback relationship between mood and reward perception. (d) Within-participant correlations between mood as estimated by the model and the participant’s self-reported feeling. The mean correlation (Pearson’sr=0.31; solid line) was positive (n=54,t53=4.5, P<10−5). Dashed line: s.e.m. Figure 3: Model-based analysis of experimental data using a reinforcement-learning model of mood. ( a ) Comparison of the mood model to the alternative ‘no mood’ and ‘no mood bias’ models in terms of each model’s ability to explain participants’ behaviour. Positive log Bayes factors favour the full mood model, and negative log Bayes factors favour the alternative model. Participants ( n =56) were divided into equal-sized groups using a median split on HPS score. Error bars: bootstrap 95% confidence intervals. ** P <10 −6 , * P <0.05, NS, P >0.5, bootstrap test. ( b ) Model-estimated mood bias (plotted on a log scale) as compared with HPS score. The more participants were susceptible to mood instability, as measured by the HPS, the more the reward-perception bias inferred by the model tended to the positive (that is, >1; n =56, Pearson’s r =0.3, P <0.05). ( c ) Participants’ model-estimated mood bias (log scale) was correlated with the degree to which striatal activity followed prediction error signals that are attributable to the effect of mood on perception of reward as compared with standard reinforcement learning prediction errors ( n =25, Perason’s r =0.43, P <0.05). Negative t -values reflect anti-correlation between the additional contribution of the positive-feedback model’s mood-induced biases (above and beyond the no-mood model prediction errors) and striatal activations, as would be expected for participants with a negative feedback relationship between mood and reward perception. ( d ) Within-participant correlations between mood as estimated by the model and the participant’s self-reported feeling. The mean correlation (Pearson’s r =0.31; solid line) was positive ( n =54, t 53 =4.5 , P <10 −5 ). Dashed line: s.e.m. Full size image Next, to determine individual effects of mood on reward perception, we established the value of f for each participant separately by fitting the mood model to the participant’s trial-to-trial choices. In line with our hypothesis, a stronger mood bias (that is, higher f ) was correlated with self-reported mood instability as measured by the HPS questionnaire ( n =56, Pearson’s r =0.30, P <0.05; Fig. 3b ). We then tested whether participants’ striatal prediction error signals were better predicted by a positive-feedback mood model than by the ‘no mood’ and ‘no mood bias’ models (both of which make the same predictions concerning striatal activity). To do this, for each participant, we generated two sequences of reward prediction error signals: one from the ‘no mood’ model and one from a mood model with positive feedback (that is, with f =2.1; see Methods). We then regressed the fMRI data against a design that included the ‘no mood’ model prediction errors, and the difference between the positive-feedback mood model prediction errors and the ‘no mood’ model prediction errors. The degree to which BOLD activity correlates with this difference reflects the degree to which the positive-feedback mood model accounted for additional variance in the striatal response to rewards, above and beyond the no-mood model [32] . The results showed that the degree to which the additional mood-model component accounted for striatal activity was correlated with participants’ inferred mood bias ( n =25, Pearson’s r =0.43, P <0.05; Fig. 3c ). Specifically, striatal prediction errors reflected the additional component predicted by the positive-feedback mood model in participants whose behaviour was consistent with a strong positive-feedback bias (that is, f in upper quartile (>1.3); mean GLM t -value 0.69±0.15), but not in participants whose behaviour indicated a weak or negative-feedback bias ( f <1.3; mean GLM t -value −0.04±0.14). In addition, the mood that the model inferred from participants’ choices and outcomes accorded with participants’ self-reported feeling throughout the experiment (mean Pearson’s r =0.31 , n =54, t 53 =4.5 , P <10 −5 , t test; Fig. 3d ). This match between the model-inferred mood and participants’ feeling held even when game 2, which was characterized by a relatively predictable change in feeling, was excluded from the analysis (mean Pearson’s r =0.27, n =52, t 51 =2.1 , P <0.05, t test). The model-inferred mood also predicted BOLD activity in frontal and temporal brain regions previously shown to distinguish between positive and negative mood [33] (mean GLM t -value 0.18±0.06, t 25 =3.0, P <0.01, t test). The theoretical consequence for mood instability Finally, we use the model to ask what would be the long-term results of such a positive feedback interaction between mood and valuation. Given that positive feedback is destabilizing, we specifically tested for the stability of mood over time. To isolate the effects of this feedback relationship from environmentally induced instability, we simulated repeated encounters with an outcome of value 10. Simulation results showed that with f ≤1 the true reward value of 10 was learned and eventually predicted, as mood did not bias perception of reward ( Fig. 4a ). However, when mood biased perception of reward so as to exert positive feedback ( f ≥1.2), good mood led to the subjective perception, and thus learning, of a higher reward value, eventually leading to disappointment once mood returned to baseline, which led to subsequent bad mood. Similarly, bad mood resulted in learning of a lower reward value that in turn led to positive surprises and good mood. Thus, mood and learned value oscillated, failing to converge to the true reward value ( Fig. 4b ). While these simulations were conducted with a particular set of parameters ( r =10, η v =0.1, η h =0.1), a dynamical system analysis of the model showed that oscillations are guaranteed to emerge as long as there are some prediction errors (that is, v init ≠ r ), and the biasing effect of mood is strong enough relative to the magnitude of the outcome and update rates (specifically, when ; see Methods). Moreover, similar dynamics emerged in simulations conducted with parameters that were inferred from the experimental data ( Supplementary Fig. 3 ), with different initial conditions ( Supplementary Fig. 4 ), with multiple states and random outcomes ( Supplementary Fig. 5 ), and with variants of the model in which mood was not bound to be between −1 and 1, or in which the effect of mood on reward perception was additive instead of multiplicative ( Supplementary Fig. 6 ). It should be noted, however, that fully predicted outcomes (that is, situations in which v init = r ) are not sufficient for oscillations to emerge. Rather, unexpected changes in outcomes are necessary, with the resulting prediction errors acting as triggers that lead to the emergence of mood instability ( Supplementary Fig. 7 ), in agreement with observational studies of bipolar patients [34] , [35] . 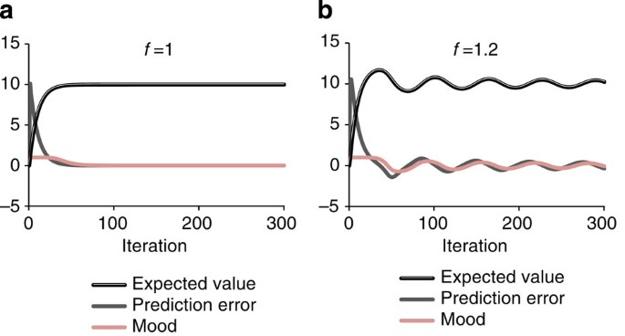Figure 4: Simulations of the interaction between learning and mood using a reinforcement-learning model. The model was repeatedly exposed to the same outcome ofr=10 for 500 iterations for each setting off, the parameter mediating the effect of mood on perception of reward. (a) Withf=1 (no mood bias), the expected value converged quickly to the true value and mood remained stable. (b) Withf=1.2 (perceived reward positively biased by mood), learned value as well as mood oscillated and did not converge. Figure 4: Simulations of the interaction between learning and mood using a reinforcement-learning model. The model was repeatedly exposed to the same outcome of r =10 for 500 iterations for each setting of f , the parameter mediating the effect of mood on perception of reward. ( a ) With f =1 (no mood bias), the expected value converged quickly to the true value and mood remained stable. ( b ) With f =1.2 (perceived reward positively biased by mood), learned value as well as mood oscillated and did not converge. Full size image Thus, mood instability emerges in a wide class of models in which unexpected outcomes affect emotional state and emotional state affects perception of outcomes, creating a positive feedback loop. It is important to note, however, that while this class of models provides a parsimonious explanation for our experimental data, there could be alternative explanations that do not involve the effect of mood. In particular, the effect of winning the WoF draw could, in principle, be explained by an accelerating (that is, convex) utility function in the domain of gains. This explanation, however, proposes a utility function that is counterintuitive and contradictory to a large body of behavioural economic research [36] , and it leaves open the question of why only high-HPS participants would have a convex utility function. Nevertheless, to establish that mood does indeed destabilize as a result of the process that our experimental and theoretical findings suggest, the effect of outcomes on mood would have to be assessed in response to multiple, successive mood-affecting outcomes. Finally, we note that it is not necessary for mood itself to affect perception of reward for our theory to explain mood instability. Instead, unexpected outcomes can affect mood as well as bias perception of subsequent outcomes. Thus, perceived outcomes could form the same unstable positive-feedback dynamics illustrated in our model, and these dynamics could lead to mood instability due to the separate effect of outcomes on mood. We thus propose our model as a candidate framework for studying disorders of mood instability. As shown above, the model can account for a cyclical pattern of mood change, as observed in psychiatric conditions such as cyclothymia and bipolar disorder [37] . In real life, mood cycles typically unfold over months [38] , [39] , [40] , [41] , making it difficult to study the full oscillatory dynamics in a laboratory experiment. However, our model provides a tool for simulating such cycles based on easily attainable information regarding the strength of a mood-valuation bias in a specific individual. This can be used to generate predictions concerning future mood dynamics, for instance, the frequency of mood cycles (for example, in the case of the rapid cycling variant [37] ), or the relationship between the timing and duration of different treatment options and their efficacy [42] . In any case, targeted, longitudinal studies of patients would be necessary to determine whether this interaction between mood and learning indeed constitutes the neuro-computational process that underlies cyclical fluctuations of mood in psychiatric conditions. Participants Thirty-one participants (mean age 21.4, age range 18–33, 25 females) performed the behavioural experiment and 33 different participants (mean age 20.6, age range 18–26, 21 females) performed the fMRI experiment. Sample sizes were determined in line with our previous experience studying across-participant correlations of behaviour, fMRI and personality measures [43] . Specifically, 30 participants, divided into two groups of 15, allow detection with a confidence level of 95% of a difference between a positive and a negative correlation that each equal r =±0.38 or higher. Participants were from the Princeton University area and gave written informed consent before taking part in the study, which was approved by the university’s institutional review board. Participants in the behavioural experiment received monetary compensation according to their performance on the task ($14.25-$32.25, mean $23.21). fMRI participants received monetary compensation for their time ($30), as well as a bonus according to their performance ($14.75-$32, mean $23.4). Stimuli All visual stimuli were designed in the processing programming environment [44] . To minimize luminance-related changes in pupil diameter, stimuli were made isoluminant with the background, to best approximation, by scaling all colours so as to equate the mean estimated perceived luminance with the background. Perceived luminance was estimated by conversion of each pixel’s RGB values from standard RGB colour space to the CIE 1976 L*a*b* space [45] . Sound effects were obtained from www.freesound.org . Slot-machine games Participants played three slot machine games, each involving three different slot machines (nine machines overall). Each machine had a distinct colour and a distinct pattern depicted on it, and some fixed probability of yielding reward when chosen. Unbeknownst to participants, within each game these probabilities were always 0.2, 0.4 and 0.6. On each trial, participants chose between two machines that appeared on the screen, and were either rewarded with 25 cents or not rewarded, according to the probability associated with the chosen machine. Participants had 3 s to make their choice. Participants’ choices were followed by a short (3.1 s) animation sequence coupled with appropriate sound effects, in which the handle of the chosen machine moved and its wheels rolled until the outcome was revealed. A ‘win’ outcome was indicated by the appearance of $ signs coupled with a metal ‘ping’ sound, whereas a ‘no win’ outcome was indicated by the appearance of X signs. The outcome stayed on the screen for 2.5 s. Inter-trial intervals were varied randomly (uniformly) between 7 and 9 s. Each game consisted of 42 trials. After the 7th, 21st and 35th trials, participants responded to the question ‘how do you feel right now?’, by choosing one out of a series of figures whose face varied from unhappy to happy (the self-assessment manikin [46] ). After the 14th, 28th and 42nd trials, participants were asked to estimate how likely each of the three slot machines in the current game was to yield reward, between 0 and 100%. Wheel of fortune To generate a large prediction error aimed at affecting participants’ emotional state, we held a single WoF draw between the first and second slot-machine games. The possible outcomes, a win or loss of $0-$8, were depicted on the wheel, which rolled, slowing down gradually, for 42 s. When the wheel stopped, an indicator above it pointed to the outcome of the draw. The rolling of the wheel and the outcome were accompanied by appropriate sound effects. Unbeknownst to participants, the draw was set up so that half of the participants won $7 and half lost $7. Participants were notified in advance that they would be paid according to their earnings in the whole experiment. There was no extra compensation to participants who lost in the WoF draw, so this loss was a real one. Test slot-machine game To compare between the valuations that participants formed in different slot-machine games, and specifically, whether the change in emotional state due to the WoF draw affected their valuations, we had participants play a final test game that involved all nine machines previously encountered. This time, however, the outcomes of choices were not shown, so that participants had to rely on what they had learned in previous games. To encourage participants to try to choose the most rewarding machines, participants were informed that ‘wins’ would be tallied towards their overall earnings, and that each slot machine ‘win’ would be rewarded with double the regular amount (that is, 50 cents). We were particularly interested in choices between slot machines that had similar reward probabilities but were encountered in different games. Thus, the test game included two trials with each such pair of machines (18 trials total). Eighteen additional trials involved pairs of machines with different reward probabilities. Of these latter trials, performance on those trials that involved one of the machines that had the highest reward probability (which we expected participants to recognize if they performed the task well) was examined to verify that participants were attentive and that they understood the task correctly. Data from one participant in the behavioural study and seven participants in the fMRI study, who did not perform above chance in the test game ( P >0.1, one-tailed binomial test) were excluded from further analysis. Questionnaires All participants filled out the international personality item pool [13] (IPIP) version of the HPS [14] . To make sure that the results reflected neither an effect of the WoF draw on responses to the HPS questionnaire, nor the reverse effect, of the HPS questionnaire on performance in the experiment, the questionnaire was administered after the WoF draw in the behavioural experiment, but before the beginning of the experiment in the fMRI experiment. In addition, to mitigate a possible recency effect on choices in the final test game, we separated in time the second and third games, as well as the third and test games, by having participants fill out additional questionnaires, whose results were not analysed. These included the BIS/BAS scales [47] , and the IPIP version of the NEO Personality Inventory [48] . Finally, to verify that the results involving HPS scores did not simply reflect the association between HPS and extraversion [15] , the results of all correlation and covariance analyses involving HPS scores were replicated after regressing out extraversion scores from HPS scores. Pupillometry A desk-mounted SMI RED 120 Hz eye-tracker (SensoMotoric Instruments, MA) was used to measure participants’ left and right pupil diameters at a rate of 60 samples per second while they were performing the behavioural task with their head fixed on a chinrest. An SMI iViewX MRI-LR unit was used to measure pupil diameter during the functional MRI experiment. Pupil diameter data were processed to detect and remove blinks and other artefacts. For each trial, baseline pupil diameter was computed as the average diameter over a period of 1 s before the beginning of the trial (at the end of the inter-trial interval, at which point pupil dilation from the previous trial should have subsided). Baseline pupil diameter measurements in which more than half of the samples contained artefacts were considered invalid and excluded from the analysis. Only participants with at least 40 valid trials were included in the pupil diameter analysis ( n =25 for the behavioural experiment, n =20 for the imaging experiment). fMRI data acquisition and preprocessing Functional (EPI sequence; 37 slices covering whole cerebrum; resolution 3 × 3 × 3 mm 3 with no gap; repetition time (TR) 2.0 s; echo time (TE) 28 ms; flip angle 71°) and anatomical (MPRAGE sequence; 256 matrix; 0.9 × 0.9 × 0.9 mm 3 resolution; TR 2.3 s; TE 3.08 ms; flip angle 9°) images were acquired using a 3T Skyra MRI scanner (Siemens, Erlangen, Germany). Data were processed using MATLAB and SPM8 (Wellcome Trust Centre for Neuroimaging, UCL). Functional data from one participant contained unusually extensive dropout artefacts in much of the brain including the striatum and were thus excluded from further analysis. Functional data were motion corrected prospectively during scanning and retrospectively using SPM. Low-frequency drifts were removed with a temporal high-pass filter (cutoff of 0.0078 Hz). The data were spatially smoothed using an 8-mm FWHM Gaussian kernel. Images were normalized to Montreal Neurological Institute (MNI) coordinates. MNI coordinates provided by the MNI space utility ( http://www.ihb.spb.ru/~pet_lab/MSU/MSUMain.html ), which correspond to the Caudate and Putamen labels in the Talairach atlas ( www.talairach.org ), were used to restrict analysis to grey matter within the striatum. General linear model We used a general linear model (GLM) to examine striatal response to reward in the different slot-machine games. The model included regressors indicating stimulus onset, response onset, ‘reward’ outcome and ‘no reward’ outcome, separately for each slot-machine game, as well as stimulus onset and response onset regressors for the rating trials. These regressors were convolved with SPM’s default hemodynamic response function. In addition, regressors of no interest reflecting head movement parameters were included in the model. As we were interested in examining activity in reward-sensitive areas of the striatum, analysis was restricted to a functional region of interest (fROI) that included all grey-matter voxels within the striatum that responded more to ‘reward’ outcomes than to ‘no reward’ outcomes throughout the experiment, according to a group-level analysis ( P <0.0001 uncorrected; similar results were obtained defining the fROI with FWE correction for multiple comparisons within the striatum ( P <0.05)). We then examined activity within this striatal fROI in response to ‘reward’ outcomes in the second game (which came immediately after the WoF draw) compared with the first game (that occurred immediately before the WoF draw). The resulting t -values were averaged across voxels within the fROI, and regressed against HPS score, WoF outcome, and the interaction between the two, using both the standard ANCOVA analysis and a more conservative robust regression analysis [26] , [27] , which accounts for potential outliers by assuming non-Gaussian noise. As a control, to test whether the WoF draw generally biased neural response to the task, we compared response to onset of the stimuli in the second game compared with the first game, in voxels that were responsive to stimulus onset according to a group-level analysis ( P <0.0001 uncorrected). This latter analysis was conducted on the whole brain, and then repeated in each cortical lobe separately, as well as in the striatum, to test for a more localized bias in the BOLD response to the task. Reinforcement learning model In standard reinforcement learning, the expected value ( v ) of a stimulus is updated according to a reward prediction error ( δ ), which reflects the difference between the actual reward obtained ( r ) and the expected value (i.e., δ = r – v ). This simple framework has proved successful in explaining a wide range of behavioural and neural data, including, most importantly, the activity of the midbrain dopamine system, which is thought to signal reward prediction error [49] , [50] . To account for effects of mood on valuation, we modified the model to compute prediction errors with respect to perceived reward rather than actual reward: where perceived reward ( r perceived ) was different from actual reward ( r ) in that it reflected the biasing effect of mood ( m ): Here, m indicates good (0< m <1) or bad (−1< m <0) mood, and f is a positive constant that indicates the direction and extent of the mood bias. If f =1 mood does not bias the perception of reward. With f >1, mood exerts positive feedback as reward is perceived as larger in a good mood and as smaller in a bad mood. Conversely, 0< f <1 corresponds to negative feedback, as reward is perceived as smaller in a good mood and as larger in a bad mood. The biasing effect of mood on reward perception was modelled as a multiplicative effect so as to maintain scale invariance [51] . We note, however, that this choice was not essential, as the same results were obtained by modelling the effect of mood on reward perception as an additive effect. To model the effects of unexpected outcomes on mood [3] , we assumed that mood reflects recent prediction-error history ( h ), tracked using a step-size parameter η h , and constrained to the range of −1 to 1 by a sigmoid function: Apart from these modifications, we assumed traditional reinforcement learning, that is, expected values were updated after every trial according to the reward prediction error with a step size (learning rate) parameter η v : The model was repeatedly exposed to an outcome of r =10 for 500 iterations. Expected value ( v ) and mood ( m ) were initialized as 0. The simulation was repeated with different values of the parameter f , which controls the degree to which mood biases perception of reward. Model-based behaviour analysis We used the mood model described above to characterize each participant’s trial-to-trial choices. In the model, a Softmax function was used to derive choice probabilities from the expected values of the available slot machines, so that the probability P ( c t = c , t ) of choosing slot machine c at trial t was proportional to . The inverse temperature parameter β controlled the exclusivity with which choices were directed towards higher-valued options. Thus, the mood model included four free parameters: f, η h , η v and β . We estimated the parameters of the model for each participant individually by computing a weighted mean of 1,000,000 randomly sampled parameterizations (importance sampling [52] ), in which each sample was weighted by the likelihood that it assigned to the observed sequence of choices, . Values v c,t were computed using the models and the preceding sequence of actual observed choices c 1… t –1 and rewards r 1… t –1 . The step-size parameters ( η h and η v ), and the inverse temperature parameter ( β ) were sampled from a uniform distribution between 0 and 1, and between 0 and 20, respectively. To avoid biasing the mood model in favour of or against a mood-consistent bias, we sampled the reward perception parameter ( f) in the log domain from a uniform distribution between ln1/10 and ln10. In addition, we compared the mood inferred by the model, based on participants’ choices and outcomes, with participants’ rating of their feeling. For this purpose, we computed for each participant the correlation between his or her nine feeling self-reports (three self-reports per game) and the mean of the model-inferred mood for each third of each game. Finally, to test whether our main results might be explained by an effect of the WoF outcome on the balance between exploration and exploitation, rather than by an effect on mood, we fit the ‘no mood’ model to participants’ choices in game 1 (before the WoF draw), and, separately, to participants’ choices in game 2 (after the WoF draw). We then repeated the analyses of test game choices and striatal responses to reward with the inclusion of a control covariate that reflected the change in the inferred inverse temperature parameter ( β ) from game 1 to game 2. Model comparison We compared the mood reinforcement-learning model, which is described above, with two alternative models: the first ‘no mood’ model is similar to the full model except that outcomes do not affect mood, which thus stays neutral (that is, equals 0) throughout the experiment. The second ‘no mood bias’ model does include an effect of outcomes on mood that is similar to the full model, but does not include an effect of mood on perception of outcomes (that is, the parameter f is set to 1). We assumed Gaussian noise on self-reports, and thus we computed the probability of observing a particular self-reported feeling given a particular model as proportional to , where m reported is the z -scored feeling reported by the participant, and m model is the z -scored mood predicted by the model at the time of self-report. We compared between the full mood model and the alternative models in terms of the likelihood that they assigned to each participant’s data, as measured by the log of the Bayes factor [53] , which was approximated by the mean log likelihood of each model given 1,000,000 random parameterizations. Since log Bayes factors were not normally distributed ( n =56, ‘no mood’ model: P <10 −14 ; ‘no mood bias’ model: P <0.005; one-sample Kolmogorov-Smirnov test [54] ), we used bias-corrected and accelerated bootstrapping [55] (with 1,000,000 samples) to estimate significance. Model-based fMRI analysis To generate model-based regressors for the imaging analysis, both the mood model and the ‘no mood’ model were simulated using each participant’s actual sequence of rewards and choices to produce per-participant, per-trial estimates of the reward prediction error signals δ t . To provide an interpretable measure for between-participant comparison, we used the same exact models to generate fMRI regressors for all participants, by instantiating each of the models with the group mean estimated parameters. Using the group mean parameters has the additional advantage of regularizing the individual estimates, which are otherwise noisy [32] , [56] . To test whether striatal activity was biased in line with a positive feedback effect of mood on reward perception, we instantiated the mood model using the mean mood bias and mood step-size parameters of participants whose mood bias parameter was consistent with positive feedback (that is, f >1). To examine the effect of mood on prediction error signals, we decomposed the series of prediction-error signals generated by the mood model into the sum of the prediction-error signals generated by the ‘no mood’ model and an additional component attributable to the effect of mood. We then used and as modulatory regressors in a GLM, which included in addition regressors for stimulus onset and choice onset, for both choice and rating trials, as well as regressors that reflect head movement parameters. We note that while and were, as expected, strongly correlated ( n =25, mean Pearson r =0.96, t 24 =10.1, P <10 −10 , t test), and were not significantly correlated ( n =25, mean Pearson’s r =−0.29, t 24 =−1.4, P =0.18, t test). Moreover, linear regression does not assign variance that is shared between two correlated regressors to either of the regressors. Thus, the GLM coefficients only reflect variance that is unique to each regressor. We verified that the striatal ROI significantly correlated with the regressor ( n =25, t 24 =7.1, P <10 −7 , t test). The t -values computed for the regressor then indicated for each participant whether the striatum demonstrated a pattern of activity that is captured by the positive-feedback mood model, above and beyond the standard model. Habel et al . [33] found nine cortical areas (excluding cerebellum, which we did not scan) that distinguished between positive and negative mood, evoked using a standardized mood-induction procedure. To test whether the mood inferred by the model matched activity in these brain areas, we created a single ROI composed of the nine corresponding spheres, which included all grey-matter voxels within a 5 voxel radius from the reported locations. We then conducted a GLM analysis, similar to the one described above, with the addition of a parametric regressor reflecting the changes in mood that were inferred by the model for each participant during the three slot machine games (the regressor was inverted for those spheres in which Habel et al . reported that activity was inversely related to positive mood). BOLD responses to this regressor were used to assess the degree to which the model-predicted mood matched activity in the ROI. Dynamical system analysis By substituting [57] δ , r perceived and m in equations 3 and 5 with the corresponding expressions in equations 1, 2 and 4, the model can be reduced to the following two-variable dynamical system: Given that the model’s update rates ( η h and η v ) have nonzero values, Δ h and Δ v both equal zero only when h =0 and v = r . Thus, the system’s only fixed point is reached when expected value is equal to the actual reward and mood is neutral. To examine whether the system is stable around this fixed point, we derived the eigenvalues ( λ ) of its Jacobian matrix: When , λ is complex and its real component equals 0, which indicates non-converging oscillations around the fixed point. With greater values of f , the real component of λ is positive, indicating that the system moves away from the fixed point. In addition, we know that the system remains bounded, given that η v <1 and η h <1, we can conclude from equations 6 and 7 that | v | cannot exceed r · f and | h | cannot exceed 2 r · f . Thus, for , the system does not approach the fixed point, but rather, continues to fluctuate within a bounded region. Simulations of the model with different values of f , r , η v and η h confirmed that is a critical value of f , beyond which the system oscillates continuously. Statistical analysis Statistical analysis was carried out using MATLAB. We did not find a significant difference between the behavioural and fMRI groups with respect to any of the effects of interest, and thus data from both experiments were pooled together where appropriate. Correlation values reported are Pearson correlation coefficients. Robust regression was performed using default options (bisquare weighting, tuning constant 4.685). Since the parameter f is multiplicative, and was sampled in the log domain, means and correlations involving f were computed in the log domain. Owing to the non-additivity of correlation coefficients, averaging of correlation coefficients was preceded by Fisher r -to- z transformation and followed by Fisher’s z -to- r transformation [58] . All results of ANCOVA interaction between HPS score and WoF outcome were replicated with the inclusion of a control regressor indicating baseline self-reported mood (measured before the WoF draw). All statistical tests reported are two-tailed. How to cite this article: Eldar, E. and Niv, Y. Interaction between emotional state and learning underlies mood instability. Nat. Commun. 6:6149 doi: 10.1038/ncomms7149 (2015).